Ocean lead at the termination of the Younger Dryas cold spell The Younger Dryas (YD) cold interval is one of the most abrupt climate events of Earth’s recent history. The origin of this rapid, severe cooling episode is still widely debated, but it was probably triggered by a large freshwater influx to the North Atlantic resulting in disruption of the Atlantic Meridional Overturning Circulation. The YD termination, despite having been even more abrupt than the onset has, however, received significantly less attention. Here using multi-proxy data from a high-resolution marine sediment record, we present evidence for a gradual decrease of the Labrador Current influence, northward migration of the Gulf Stream oceanic front and a rapid decline of sea-ice cover at the YD termination. Our data indicate a stepwise sequence of events with changes in ocean circulation clearly preceding those in atmospheric conditions, in contrast to the hitherto commonly assumed single-event rapid climatic shift at the YD–Holocene transition. The Younger Dryas (YD) was a major climatic event during the transition from the last glacial period into the present Holocene interglacial. During approximately 1,200 years [1] , the deglacial warming was paused and the North Atlantic region returned to near-glacial conditions, with a major impact on global climate [2] , [3] , [4] . Most probably caused by a large freshwater influx to the North Atlantic [5] , [6] , [7] , a slowdown of the Atlantic Meridional Overturning Circulation (AMOC) resulted in a reduction of northward heat transport. The intensity of the AMOC regulates to a large extent the heat transport from the tropics to higher latitudes and has played an important role in abrupt deglacial climate changes [8] . During the YD cold interval, a southward shift of the Gulf Stream (GS)—North Atlantic Current system ( Fig. 1 ) resulted in a decrease of the overturning intensity and caused a widespread cooling in the North Atlantic region. The abrupt warming following the YD has been associated with a rapid acceleration of the AMOC after centuries of reduced intensity [8] . However, there is still limited understanding of the parameters driving the change in the overturning intensity and the rate at which these events have occurred. 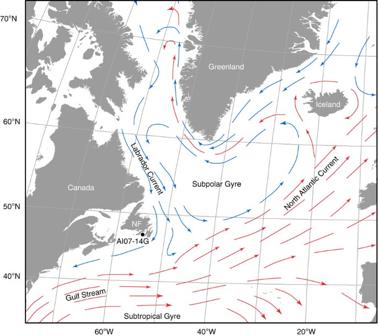Figure 1: Map of the study area with location of marine sediment core AI07-14G. The map shows ocean gyres and major surface currents. Red arrows: warm-water currents; blue arrows: cold-water currents. NF, Island of Newfoundland. Figure 1: Map of the study area with location of marine sediment core AI07-14G. The map shows ocean gyres and major surface currents. Red arrows: warm-water currents; blue arrows: cold-water currents. NF, Island of Newfoundland. Full size image The coastal waters off southeastern Newfoundland represent an ideal location for studying past AMOC variability. Influenced by water masses from the cold Labrador Current (LC) and the warmer and more saline GS waters, the area is currently situated at the oceanic front between the North Atlantic Subpolar Gyre and the Subtropical Gyre ( Fig. 1 ). The area is also located in the atmospheric frontal zone between cold polar air masses and warmer air from the south [9] . Previous studies from the region have shown a ca. 10 °C warming of surface waters south of Newfoundland [10] , as well as a rapid response of the terrestrial vegetation [11] to the warming during the YD–Holocene transition, but the temporal resolution of these records did not allow for accurately determining the rate of these changes. In this study, we present results from a multi-proxy analysis of a marine sediment core from Placentia Bay, Newfoundland ( Fig. 1 ), which spans the YD–Holocene transition at high temporal resolution. Our data show a gradual warming in the western North Atlantic in the final stage of the YD, followed by a rapid decline of sea-ice concentrations and deposition of a detrital carbonate layer associated with Heinrich event 0 (H0), possibly linked to the rapid termination of the YD found in the NGRIP (North Greenland Ice Core Project) ice core and Cariaco Basin marine sediments [1] , [12] , [13] . Data interpretation Our reconstruction of the sequence of events at the YD termination is based on the analysis of marine sediment core AI07-14G from 239 m water depth in Placentia Bay, Newfoundland ( Fig. 1 ). The age of the core ranges from ca. 10–13 kyr BP (thousand years before present, defined as AD 1950) with an average chronological resolution of 6.3 years cm −1 ( Fig. 2 ), allowing the study of the YD–Holocene transition at a sub-decadal temporal resolution. The core was investigated using a multi-proxy approach consisting of sedimentological, micropaleontological and geochemical analyses ( Fig. 3 ). The Ca/Sr ratio, calculated from X-ray fluorescence core scan measurements, was used to identify the presence of a peak in detrital carbonate, associated with H0 around 11.6 kyr BP [14] , [15] , [16] . The presence of H0 was confirmed by X-ray diffraction (XRD) analyses, which showed increased concentrations of calcite and dolomite within the carbonate peak, characteristic of H0 sediments [17] . Fossil diatom assemblages were used to infer past surface-water conditions and provide information on the relative influence of the main ocean currents. Thalassiosira gravida , an arctic cold-water diatom species, documents the influence of the LC, whereas the warmer-water species Thalassionema nitzschioides was used to track the influence of GS waters [18] , [19] . The abundance of IP 25 , a biomarker synthesized by diatoms living in sea ice [20] , [21] , was measured to reconstruct past variability in spring sea-ice cover. 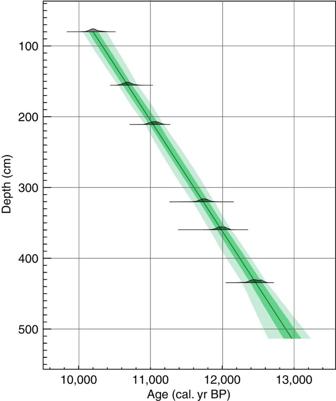Figure 2: Age-depth model for core AI07-14G. The model starts from 78 cm depth in the core and is based on six radiocarbon measurements (Table 1). Light and dark green areas illustrate the 68% and 95% probability range, respectively. cal. yr BP, calibrated years before present. Figure 2: Age-depth model for core AI07-14G. The model starts from 78 cm depth in the core and is based on six radiocarbon measurements ( Table 1 ). Light and dark green areas illustrate the 68% and 95% probability range, respectively. cal. yr BP, calibrated years before present. 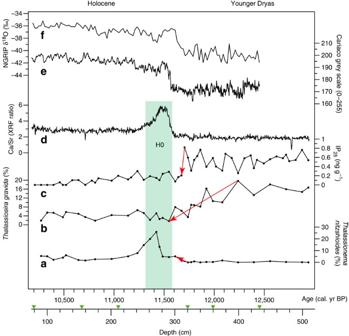Figure 3: Results from core AI07-14G and comparison with the NGRIP and Cariaco records. (a) Relative abundance of the warm-water diatomT. nitzschioides. (b) Relative abundance of the cold-water diatomT. gravida. (c) Abundance of the sea-ice biomarker IP25. (d) Calcium/strontium ratio (Ca/Sr) from X-ray fluorescence (XRF) core scanning. (e) Grey scale from Cariaco basin core PL07-56PC12. (f) Stable oxygen isotope δ18O profile from the NGRIP ice core1. Green triangles show the position of samples analyzed for radiocarbon. Red arrows indicate major shifts in the different proxies discussed in the text. Green shading indicates the position of H0 sediments. cal. yr BP, calibrated years before present. Full size image Figure 3: Results from core AI07-14G and comparison with the NGRIP and Cariaco records. ( a ) Relative abundance of the warm-water diatom T. nitzschioides . ( b ) Relative abundance of the cold-water diatom T. gravida . ( c ) Abundance of the sea-ice biomarker IP 25 . ( d ) Calcium/strontium ratio (Ca/Sr) from X-ray fluorescence (XRF) core scanning. ( e ) Grey scale from Cariaco basin core PL07-56PC [12] . ( f ) Stable oxygen isotope δ 18 O profile from the NGRIP ice core [1] . Green triangles show the position of samples analyzed for radiocarbon. Red arrows indicate major shifts in the different proxies discussed in the text. Green shading indicates the position of H0 sediments. cal. yr BP, calibrated years before present. Full size image The YD to Holocene transition High concentrations of T. gravida and IP 25 reveal that the YD interval was characterised by a major influence of the cold LC bringing heavy sea-ice conditions ( Fig. 3 ). Contrasting with these cool but stable conditions during the main part of the YD, the transition into the warmer Holocene shows rapid changes in sea surface conditions and oceanic circulation. These are recorded in the different proxy records as a clear stepwise sequence of events. The first indication of the YD termination is a gradual decrease in the relative abundance of T. gravida , reflecting a progressive reduction of the LC influence in the area, which started as early as ca. 12.2 kyr BP ( Fig. 3b ). At the same time, concentrations of IP 25 start showing stronger variability, indicating the initiation of unstable sea-ice conditions. Around 11.7 kyr BP, a slight increase in the warmth-indicating diatom species T. nitzschioides ( Fig. 3a ) suggests a gradually increased influence of the warm, high-energy GS. The northward migration of the oceanic front and therefore the enhanced transport of heat to the area resulted in a concurrent, sharp (within 50 years) decrease in sea-ice cover at around 11.7 kyr BP ( Fig. 3c ). Starting at 11.6 kyr BP, Ca/Sr ratios peak abruptly ( Fig. 3d ) as the result of input of detrital carbonate originating from H0 hypopycnal plumes in the surface waters on the shelf. During deposition of the H0 detrital carbonate layer, concentrations of T. nitzschioides show an abrupt, but short-lived increase as a result of the release of nutrients associated with the H0 plume. During the Holocene, conditions are generally more stable with low sea-ice concentrations and decreased influence of the LC. Chronologies based on marine radiocarbon dating always have inherent uncertainties, based on both the errors associated with the calibration itself and the uncertainties in the local marine reservoir age. Therefore, uncertainty ranges in the age determination of a single depth in core AI07-14G can be as high as several centuries ( Fig. 2 and Table 1 ). However, because all the proxy records used for our palaeoenvironmental reconstruction ( Fig. 3a–d ) are derived from one single sedimentary archive, any potential age offsets between events leading up to the YD termination can be excluded. It can therefore be stated that the termination of the YD was not a single shift but rather a succession of distinct, temporally separated events, initiated by changes in the oceanic circulation pattern. Table 1 Radiocarbon dates and calibrations from core AI07-14G. Full size table Based on our reconstructions, we suggest the following sequence of events leading up to the YD termination. Over the later part of the YD period (ca. 12.3–11.7 kyr BP), the influence of the LC gradually decreased and the GS-LC oceanic front migrated northwards. This northward movement of the frontal zone, probably linked to AMOC picking up in strength [8] , led to more unstable sea-ice conditions as inferred from the highly variable IP 25 concentrations ( Fig. 3c ) and coincides with results from other studies also indicating a contrast between a stable early YD and an unstable late YD [22] . Just before H0 and the YD termination, our record shows a rapid loss of sea-ice cover and an increased influx of warmer GS source waters, centuries after the initial decline in LC influence. Because these gradual and more abrupt transitions pre-date the occurrence of H0 in the record, they must also pre-date the YD–Holocene transition, as H0 has been shown in a number of studies to occur within the YD [14] , [15] , [16] , [17] . Rapid shifts in climate (atmospheric conditions) at the YD–Holocene transition have previously been recorded from other high-resolution records from both high and low latitudes of the North Atlantic region. Greenland ice core records [23] , [24] illustrate variations linked to shifts in the atmospheric Polar Front within 50 years, whereas in the tropics, a northward shift in the Intertropical Convergence Zone (ITCZ) is a prominent feature of the YD–Holocene transition [13] , [25] , [26] . Despite the limitations inherent in marine 14 C age models, it is clear from our record that the reduction in the LC influence and the northward migration of the oceanic front occurred before the H0 event and thus pre-date the end of the YD. The observed warming in the western North Atlantic as the result of changes in ocean circulation thus unambiguously occurred before the atmospheric shift recorded in the Greenland ice sheet and Cariaco basin, associated with the onset of the Holocene. Hughen et al . [25] suggested that the stronger trade winds over the Cariaco basin region during the YD probably derived from a cold, ice-covered northern North Atlantic and a more southerly location of the ITCZ. Similarly, other studies suggested a general link between cold Greenland winters, strong trade winds, a southern ITCZ position and a weaker GS [27] . Finally, Talbot et al . [26] linked a sudden trade wind weakening at the end of the YD to shifts in the bipolar seesaw [28] . This suggests that the changes in ocean circulation leading up to the YD termination from our data set may also be linked to changes in the tropics and the southern hemisphere and may, in fact, be the trigger of the general northward shift of both the ITCZ and the atmospheric polar front observed at the YD/Holocene transition [13] , [24] . It has already been hypothesized that ocean circulation in the North Atlantic may have had major influence on the YD–Holocene climate transition [25] and that the ocean may lead the atmosphere during periods of major glacial to interglacial climate transitions [29] . The present study provides, however, the first unambiguous evidence of such an ocean lead for the YD–Holocene transition, a result which can be of great value to the climate modelling community and the projection of future climate scenarios. Our data suggest that North Atlantic ocean circulation has, in fact, an even greater role at times of rapid climate change than previously assumed, also supporting model studies that indicate a very sensitive AMOC system today [30] , [31] . Coring Marine sediment core AI07-14G was obtained using a gravity corer from aboard the Russian research vessel ‘Akademik Ioffe’ on 27 September 2007. The core consists of 513.5 cm of marine silty clay and was retrieved from 239 m water depth in Placentia Bay (46°59.327′N, 54°42.046′W; Fig. 1 ). In the laboratory, the core was split and stored at 3 °C. One half was kept intact as an archive, whereas the ‘working’ half was sampled at regular intervals for sedimentological, geochemical and micropaleontological analyses. Chronology To establish a chronology for the core, seven samples were measured for radiocarbon content at the AMS 14 C Dating Centre of Aarhus University, Denmark ( Table 1 ). Samples consisted of marine mollusks ( Portlandia arctica and Mya truncata ), mixed benthic foraminiferal assemblages and unidentified mollusk shell fragments ( Table 1 ). The age-depth model for core AI07-14G was made using a P_Sequence depositional model in the Oxcal 4.2beta [32] , [33] software. All dates were calibrated using the Marine09 14 C calibration data set [34] using the modern day total reservoir correction age of 539±61 years [35] . The six lowermost 14 C dates are in the age range of 10–12.6 cal kyr BP, whereas the upper sample, which was taken from a sand layer at the top of the core, has a much younger age ( Table 1 ). This indicates that the sandy top layer was deposited much later than the rest of the core and may represent a lag in the sediment sequence. The origin of this is unknown, but could have been caused by several mechanisms, such as erosion, non-deposition, ice berg scouring [36] , [37] or even the 1929 Grand Banks earthquake [38] . Because the upper section holds only one radiocarbon date, and the coarser, sandy sediments may represent a reworked, lag-type deposit, the top 78 cm of the core (well below the sand layer) was excluded from further discussion in this study. Hence, the age model of core AI07-14G is based on six radiocarbon measurements starting at a depth of 78 cm ( Fig. 2 ) and has a chronological resolution of 6.36 years cm −1 . Sedimentological and geochemical analyses The geochemical composition of the sediment was analysed at 0.2 mm resolution (and subsequently stacked to 5 mm intervals) using an Itrax X-ray fluorescence core scanner (molybdenum tube) at the Department of Geoscience, Aarhus University. Using this non-destructive method, semiquantitative measurements were obtained for the various elements in the core. The Ca/Sr ratio shown in Figure 3d was calculated by dividing the measurements from Ca and Sr in counts per second. XRD bulk analyses on selected samples were performed on a PANalytical X’pert Pro MPD with Cu-K alpha radiation and Ge monochromator (40 mA and 45 kV) at the Department of Geoscience, Aarhus University. A total of 60 samples were analysed for determination of IP 25 abundances in the sediments. Samples were freeze-dried and an internal standard (7-hexylnonadecane) was added. Highly branched isoprenoids (HBIs) were extracted using a mixture of CH 2 Cl 2 /CH 3 OH (2/1), and hydrocarbon fractions were obtained from the total organic extract using open column chromatography (SiO 2 /hexane). Hydrocarbon fractions were analysed using an Agilent Technologies 7890 gas chromatograph system coupled to an Agilent Technologies 5975C inert XL mass selective detector. The gas chromatograph was fitted with a 30 m HP5MS column (0.25 mm i.d., 0.25 μm film thickness) and the oven temperature programmed from 40 to 300 °C at 10 °C min −1 and held at the final temperature for 10 min. Operating conditions for the mass spectrometer were 250 °C for the ion source temperature and 70 eV for the ionisation energy. Spectra (50–550 Da) were collected using Agilent MassHunter software. Individual HBIs were identified by comparing their retention time and mass spectral characteristics with those of previously authenticated HBIs (for example, Johns et al . [39] ). Peak area integration of selective ion monitoring chromatograms was performed to quantify the abundance of IP 25 ( m/z 350.3). HBI abundances are expressed in μg relative to the internal standard ( m/z 99.0) as ng (internal standard equivalent)/g (mass of the sediment sample). Diatoms Throughout the core, 39 samples were analyzed for diatom content. The samples were freeze-dried, and for every sample, 0.2–1 g of dry sediment was subsequently treated with a hydrogen peroxide solution (35%, 1.5 h at 100 °C) and a few drops of hydrochloric acid (37%) to remove all organic matter and carbonates, respectively. The solution was cleaned with demineralized water through a cycle of sedimentation and decantation for a minimum of five times. Microscope slides were prepared by pipetting a known concentration of the solution into sedimentation trays [40] where it could settle on cover slips. The cover slips were then mounted on the slides using the high refractive index mountant Naphrax. For each sample, at least 300 diatom valves, excluding Chaetoceros resting spores, were identified and counted at × 1,000 magnification using a Leica DMLB microscope equipped with phase contrast optics. Diatom identification followed standard taxonomical literature for marine diatoms [41] , [42] , [43] , [44] . How to cite this article: Pearce, C. et al . Ocean lead at the termination of the Younger Dryas cold spell. Nat. Commun. 4:1664 doi: 10.1038/ncomms2686 (2013).